Photocatalyzed cycloaromatization of vinylsilanes with arylsulfonylazides 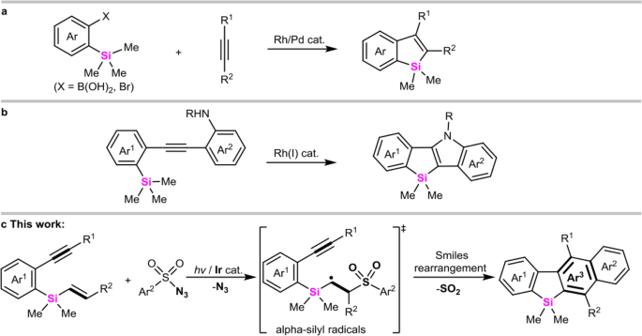Fig. 1: Strategies to access benzosiloles. aRh/Pd-catalyzed intermolecular cyclovinylation of arylalkylsilanes with alkynes.bRh(I)-catalyzed intramolecular aminosilylation ofortho-alkynylarylsilanes.cPhotocatalyzed carbocyclization of vinylsilanes with arylsulfonyl azides via alpha-silyl radical Smiles rearrangement. Sila-molecules have recently attracted attention due to their promising applications in medical and industrial fields. Compared with all-carbon parent compounds, the different covalent radius and electronegativity of silicon from carbon generally endow the corresponding sila-analogs with unique biological activity and physicochemical properties. Vinylsilanes feature both silyl-hyperconjugation effect and versatile reactivities, developing vinylsilane-based Smiles rearrangement will therefore provide an efficient platform to assemble complex silacycles. Here we report a practical Ir(III)-catalyzed cycloaromatization of ortho -alkynylaryl vinylsilanes with arylsulfonyl azides for delivering naphthyl-fused benzosiloles under visible-light photoredox conditions. The combination of experiments and density functional theory (DFT) energy profiles reveals the reaction mechanism involving α-silyl radical Smiles rearrangement. Silahydrocarbons are sometimes encountered in pharmaceuticals and material chemistry [1] , [2] , [3] , [4] . Compared with all-carbon parent compounds, Si-element generally endows the corresponding hydrocarbons with unique biological activity and physical–chemical properties [5] , [6] , [7] , [8] , which are mainly determined by the different covalent radius and electronegativity of silicon from carbon. In these regards, arene-fused siloles have especially attracted many concerns due to their promising applications in electronic and optoelectronic devices [9] , [10] , [11] , [12] , [13] . In 2012, Xi [14] and Chatani [15] pioneeringly explored intermolecular coupling-cyclization of alkynes with 2-silylaryl bromides and 2-silylphenylboronic acids to produce 2,3-difunctionalized benzosiloles through Si-C bond cleavage (Fig. 1a ). Subsequently, He [16] developed rhodium-catalyzed intramolecular silicoamination of ortho -alkynylarylsilanes to construct indole-fused benzosiloles (Fig. 1b ). In light of that modifying the π-conjugated system of parent siloles could possibly improve their corresponding photophysical properties. Thus, there has been an ever-increasing demand for the rapid assembly of diversified polycycle-fused siloles [17] , [18] , [19] , [20] , [21] , [22] . Fig. 1: Strategies to access benzosiloles. a Rh/Pd-catalyzed intermolecular cyclovinylation of arylalkylsilanes with alkynes. b Rh(I)-catalyzed intramolecular aminosilylation of ortho -alkynylarylsilanes. c Photocatalyzed carbocyclization of vinylsilanes with arylsulfonyl azides via alpha-silyl radical Smiles rearrangement. Full size image Aryl migration via Smiles rearrangement is a powerful tool for the synthesis of polycyclic arenes [23] , [24] , [25] . However, the modes of radical Smiles rearrangement are very limited. Up to now, only α-carbonyl radical [26] , [27] , [28] , [29] , [30] , β-aminoalkyl radical [31] , [32] , [33] , N -centered radical [34] , and ketyl radical [35] - triggered Smiles rearrangement have been exploited to construct nitrogen-heterocycles, and vinylsilane-based Smiles rearrangement keep unexplored. As is well known, vinylsilanes have proven to be important “alkene” sources in Hiyama coupling, which could efficiently incorporate C=C bond in a particular molecule with the release of silyl moiety [36] ; Meanwhile, the high electronegativity of carbon (2.35) relative to silicon (1.64) [37] and silyl-hyperconjugation effect (the so-called β-effect) [38] , [39] , [40] generally endow these compounds with the versatile reactivity. For example, Jun [41] reported that Rh(I)-catalyzed cross-coupling of aldehydes with vinylsilanes led to the formation of β-acylsilanes via β-silylethylrhodium(III) intermediates. On the contrary, Buchwald [42] and Miura [43] demonstrated that Cu(I)-catalyzed addition-coupling of vinylsilanes with amines could produce α-aminosilanes. Thus it can be seen that developing vinylsilane-based coupling-cyclization will possibly establish an efficient platform to assemble complex silacycles. Again, azides could be employed as potential nitrogen radical precursors to enable C-H amination [44] under photocatalysis systems. Accordingly, visible-light catalyzed coupling of vinylsilanes with arylsulfonylazides could possibly generate α -silyl radicals and initiate the silylalkene Smiles rearrangement. Here, we show a cycloaromatization of ortho -alkynylarylsilylalkenes with arylsulfonyl azides for rapid assembly of 2,3-naphthyl-fused benzosiloles via a cascade S-N/C-S bond cleavage in the presence of visible light (Fig. 1c ). Investigation of reaction conditions The choice of ortho -alkynylaryl vinylsilane 1a was motivated by the notion that alkynyl and vinyl groups could possibly trap radicals to assemble complex silacycles under blue light-emitting diodes (LEDs) irradiation. After an extensive screening of various reaction parameters, we were pleased to find that the treatment of substrate 1a with TsN 3 2a under photocatalyzed system did afford a large π-conjugated benzosilafluorene 3a with an unexpected loss of sulfonylazide (SO 2 N 3 ) group from TsN 3 (Fig. 2 ). Optimization of the reaction conditions afforded the yield of 3a reaching 69% in the presence of 0.5 mol % of [Ir{dt(tBu) 2 ppy} 2 (dtbbpy)][PF 6 ] ( PC1 ) and 1,4-diazabicyclo(2.2.2) octane (DABCO) (1.5 equiv) in 1,4-dioxane at 80 °C for 24 h under air atmosphere (Fig. 2 Table, entry 1). On the contrary, other catalysts such as fac -Ir(ppy) 3 ( PC2 ), Eosin Y, MesAcr + ClO 4 − ( PC3 ), 2,4,6-triphenylpyrylium tetrafluoroborate (TPP), and Ru(bpy) 3 Cl 2 ( PC4 ) did not give the product 3a in more than 5% yield (entries 2–6 vs 1). 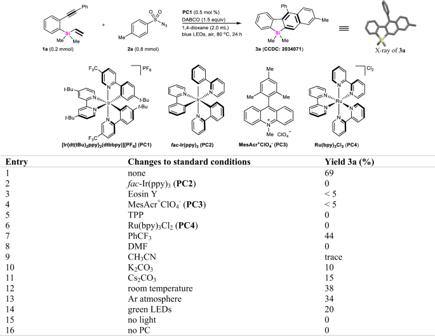Fig. 2: Reaction development. All the reactions are conducted in sealed tubes, followed by flash chromatography on SiO2. The isolated yields are reported. Meanwhile, utilization of different solvent systems (entries 7–9) or inorganic bases such as K 2 CO 3 and Cs 2 CO 3 (entries 10–11) made this transformation very sluggish. Similarly, running the reaction under room temperature, Ar atmosphere, and green-light irradiation also led to significantly lower yields, respectively (entries 12–14 vs 1). Notably, control experiments under these optimized conditions indicated that 2,3-naphthyl-fused benzosilole 3a could not be observed at all in the absence of light or photocatalysts ( PC ) (entries 15–16). Fig. 2: Reaction development. All the reactions are conducted in sealed tubes, followed by flash chromatography on SiO 2 . The isolated yields are reported. Full size image Substrate scope With this optimized protocol, we examined the transformation of various ortho -alkynylaryl vinylsilanes ( 1 ) with para -methylphenylsulfonyl azide 2a . As summarized in Fig. 3 , different sila-enynes 1 bearing electron-rich (-Me, -Et, - n -Bu, and -MeO), halogen (-F, -Cl and -Br), strong electron-withdrawing (-CF 3 ), and even vinylsilyl substituent at the para -position of alkynylphenyl groups (R 1 = phenyl), successfully underwent carbocyclization-aromatization with TsN 3 ( 2a ) to afford 4-(4-substituted-phenyl)-2,3-benzosilafluorenes 3a , 3b , 3d – 3k in moderate to good yields (50–71%). Likewise, meta -methylphenyl-substituted alkynylaryl vinylsilane could react efficiently to provide 3c in 63% yield. Meanwhile, ortho -(1-heptynyl)-phenyl vinylsilane was also tolerable in this reaction to assemble 4-pentyl-substituted-2,3-benzosilafluorenes 3l (50%). However, when the terminal alkyne-tethered arylvinylsilane was subjected to the reaction system, only a 15% yield of 3m was obtained. The evaluation of the substituent effect (R 3 ) from vinylsilyl benzene ring of 1 indicated that all of the electron-rich or electron-deficient silylarenes could smoothly react with TsN 3 ( 2a ) to furnish the desired products 3n – 3q with good conversions (58–68% yields), regardless of electronic properties of substituents. It should be noted that hept-1-en-1-yldimethylsilane was not well tolerated under these conditions, only affording 1-pentyl-2,3-benzosilafluorene 3r in 12% yield. Fig. 3: Sila-enyne scope. All the reactions are conducted in sealed tubes, followed by flash chromatography on SiO 2 . The isolated yields are reported. Full size image Interestingly, if vinyldimethylsilane 1 was switched to allyldimethylsilane 4 , an unexpected [2 + 2 + 3] coupling-cyclization of ortho -alkynyaryl allyldimethylsilane 4 with arylsulfonyl azides 2 occurred (Fig. 4 ), affording a novel 6/7/7/6-fused silatetracyclic skeleton in good yields (59–65% for 5a – 5c ) in which SO 2 was kept untouched. Fig. 4: The coupling-cyclization of allylic dimethylsilanes with arylsulfonyl azides. All the reactions are conducted in sealed tubes, followed by flash chromatography on SiO 2 . The isolated yields are reported. Full size image Next, we explored the substrate scope of sulfonyl azides by carrying out the cycloaromatization reaction with vinylsilane 1a (Fig. 5 ). Compared with electron-neutral phenylsulfonyl azides (60% for 6a ), 4-MeO, 4-Ph, 4-halo (F, Cl, Br, I), and 4-acetamido-phenylsulfonyl azides could smoothly react with vinylsilane 1a to produce 2,3-benzosilafluorenes in 21–70% yields ( 6d , 6e , 6h , 6i , 6l , 6m , 6n ). Of noted, 3-methylphenylsulfonyl azide, 3-chlorophenylsulfonyl azide, and even 2-naphthylsulfonyl azide furnished 61–74% overall yields of isomers 6b / 6c , 6f / 6g , and 6j / 6k . Gratifyingly, the protocol was still shown to tolerate strong electron-withdrawing (4-CF 3 , 4-CN, 4-acyl, 4-CO 2 Et, 4-CO 2 H) substituted phenylsulfonyl azides and even 3-pyridylsulfonyl azide, giving 42–72% yields of 6o – 6t , respectively. Fig. 5: Arylsulfonylazide scope. All the reactions are conducted in sealed tubes, followed by flash chromatography on SiO 2 . The isolated yields are reported and ratios of isomers are shown in parenthesis. Full size image Application To evaluate the potentiality of 2,3-naphthyl-fused benzosiloles in developing organic optoelectronic materials, 8-bromo-5,5-dimethyl-11-phenyl-5H-benzo[b]naphtho[2,3-d]silole 6l was employed to react with anthracene-9,10-diyldiboronic acid 7 in the presence of Pd-catalysts, and highly π-conjugated teranthracene-tethered 1-phenyl-2,3-benzosilafluorene 8 which contains three anthracenyl units, could be obtained in 14% yield (Fig. 6a ) (it should be noted that this transformation easily led to the protonation of anthracene-9,10-diyldiboronic acid 7 , affording 53% yield of anthracence 9 (see Supplementary Information, pg S26)). Photophysical properties of benzosilole derivative 8 were investigated by ultraviolet-visible (UV-vis) absorption and photoluminescence (PL) spectra in diluted toluene solution (10 −5 M) (Fig. 6b ). The absorption bands in the long-wavelength region (350–400 nm) can be attributed to the π–π* transition of the anthracenyl units [45] . Both PL spectra at r.t. and 77 K exhibited a 0–0 peak at 415 nm, a 0–1 sub-peak at 433 nm, and a 0–2 shoulder at 465 nm. Meanwhile, a PL quantum yield of 51% was achieved, indicating that this molecular skeleton could be a promising building block for deep-blue luminescent materials. Fig. 6: Synthetic applications of this method. a Synthesis of π-conjugated teranthracene-tethered 1-phenyl-2,3-benzosilafluorene 8 . b UV-vis absorption and PL spectra of benzosilafluorene 8 measured in diluted toluene solution (10 −5 M) (a.u. refers to the arbitrary unit. Fluo@298K refers to the fluorescence spectra measured at 298 K. Fluo@77K refers to the fluorescence spectra measured at 77 K. Phos refers to the phosphorescence spectra.). Full size image Mechanistic investigations Sulfonyl azides have been rarely converted into sulfonyl radicals in chemical transformation. Up to now, only Konig reported an example that sulfonyl azides were employed as precursors of nitrenes in visible-light photocatalysis [46] . More recently, Lam found that arylsulfonyl azides could be converted into arylsulfonyl radicals under the photocatalytic system, in which hydrogen abstraction from THF was involved [47] . However, our solvent screening indicated that this cycloaromatization could also be allowed in PhCF 3 (Fig. 2 , entry 7), in which hydrogen abstraction from PhCF 3 is very difficult. The observation implied that sulfonyl azides could possibly produce sulfonyl radical via unstable arylsulfonyldiimide intermediates (ArSO 2 N=NSO 2 Ar) [48] , which is derived from the nitrene radical dimerization and protonation (this transformation was performed under air conditions, in which the synergistic cooperation of O 2 , and alkylamines (DABCO), etc. could possibly provide proton sources) [49] . Given that disulfonylhydrazines could produce disulfonyldiimines via single electron transfer (SET) followed by denitrogenation to afford sulfonyl radicals [50] , [51] , we utilized sulfonylhydrazine 10 to react with 1a (Fig. 7a ), the desired product 3a (30%) could be obtained, this control experiment implied that disulfonyldiimines were possibly involved in this cycloaromatization. Fig. 7: Preliminary mechanism studies. a Photocatalyzed cycloaromatization of vinylsilane 1a with sulfonylhydrazine 10 . b Radical intermediate trapping reaction by TEMPO. c Photocatalyzed coupling-cyclization of vinylether 1u with arylsulfonylazide 2h . d Photocatalyzed coupling-cyclization of vinylsilane 1a with ortho -methylphenylsulfonyl azide 2s . Full size image In addition, when 2,2,6,6-tetramethyl-1-piperidinyloxy (TEMPO) (2.0 equiv) was applied to the reaction of vinylsilane 1a and TsN 3 , it was found that TEMPO completely inhibited the cycloaromatization of 1a , and sulfonyl ester 11 (HR-MS: 334.1448, Supplementary Fig. 3 ) (see Supplementary Information for the HR-MS) could be detected (Fig. 7b ), confirming that sulfonyl radicals were involved in this transformation. Interestingly, changing vinylsilane ( 1a ) to vinylether ( 1u ) produced a seven-membered ring compound 12 (CCDC 2034125) instead of cycloaromatization product 13 (Fig. 7c ). This experiment demonstrated that Si/O switch significantly affected the reaction pathway of vinylsilanes, in which sulfonyl radicals derived from sulfonyl azides preferred to attack carbon-carbon double bonds instead of carbon-carbon triple bonds. 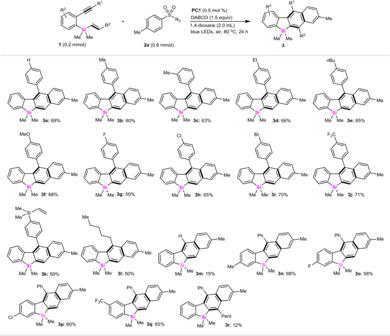Fig. 3: Sila-enyne scope. All the reactions are conducted in sealed tubes, followed by flash chromatography on SiO2. The isolated yields are reported. Furthermore, compared to para - or meta -methylphenylsulfonyl azides ( 3a in Fig. 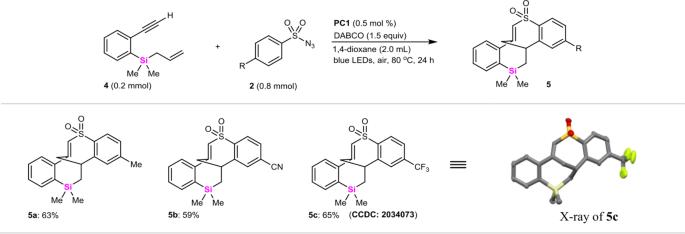Fig. 4: The coupling-cyclization of allylic dimethylsilanes with arylsulfonyl azides. All the reactions are conducted in sealed tubes, followed by flash chromatography on SiO2. The isolated yields are reported. 3 , 6b / 6c in Fig. 5 ), the coupling-cyclization of ortho -methylphenylsulfonyl azide 2s with vinylsilane 1a only afforded a 16% yield of non-aromatized silacycle 14 (CCDC 2064550), and the aromatized silacycle 6u was not obtained possibly due to that steric hindrance of ortho -methyl substituent of 2s inhibited a potential structural arrangement and subsequent aromatization (Fig. 7d ). Phosphorescence spectra of the diluted toluene solutions detected at 77 K with a delay time of 0.05 ms were employed to determine the triplet energies of PC1 (2.58 eV) and TsN 3 (3.10 eV) (Supplementary Fig. 2 ), demonstrating that an energy transfer (EnT) process between the excited state *Ir(III)-catalyst PC1 and TsN 3 could not occur. Meanwhile, the reduction potential difference (~0.39 V) between PC1 ( E III/IV : −1.45 V versus Ag/AgNO 3 in CH 3 CN) and TsN 3 ( E red : −1.06 V vs Ag/AgNO 3 in CH 3 CN) (see Supplementary Information for the cyclic voltammetry (CV) of TsN 3 and Ir(III)-catalyst PC1 ) means that the electron transfer between them possibly occurred under heating conditions (Supplementary Figs. 4 and 5 ). 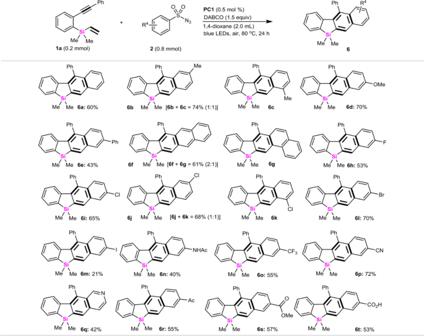Fig. 5: Arylsulfonylazide scope. All the reactions are conducted in sealed tubes, followed by flash chromatography on SiO2. The isolated yields are reported and ratios of isomers are shown in parenthesis. Moreover, the fluorescence quenching (Supplementary Figs. 6 and 7 ) further suggested that a possible SET process between the excited state *Ir(III)-catalyst and TsN 3 led to the formation of sulfonyl radicals via nitrene radicals [52] and arylsulfonyldiimide [48] . Calibrated with DFT calculations, the possible reaction mechanism is shown in Fig. 8 . In Path a, the addition of sulfonyl radical to the carbon-carbon double bond in substrate 1a results in α-silyl carbon radical A (5.6 kcal/mol), which could further undergo the radical cyclization with carbon-carbon triple bond to afford vinylradical B (−11.6 kcal/mol). Intramolecular cyclization of B at the benzene ring followed by the Smiles rearrangement involved a spirocyclic intermediate C (−12.7 kcal/mol) and a subsequent desulfonylation to produce beta-silyl radical D (−29.9 kcal/mol). Again, the cascade radical cyclization to E (−41.4 kcal/mol), SET, and aromatization give the cycloaromatization product 3a . In contrast, Ts• radical could attack the carbon-carbon triple bond of 1a in Path b, leading to ethylenic radical G (8.0 kcal/mol), which then forms radical intermediate H (−2.0 kcal/mol) and I (−4.8 kcal/mol) through cascade cyclization. Although intermediate I could be converted to E by desulfonylation, control experiments and DFT calculations both suggest Path a to be the more plausible mechanism. Because of that ortho -methylphenylsulfonyl azide 2s was subjected to the standard photocatalyzed system, although ortho -methylphenylsulfonyl radical could attack the carbon-carbon double bond of 1a , the steric hindrance from ortho -methyl substituent of 2s possibly inhibited the formation of the spirocyclic intermediate C (Path a), resulting in very poor yield (16%) of non-aromatized silacycle 14 (see Supplementary Information for the HMBC, NOE spectra and single crystal structure (Supplementary Figs. 8, 9, and 15) of compound 14 ) through cascade radical cyclization and desulfonylation. This control experiment (Fig. 7d ) indirectly implied that the cycloaromatization between vinylsilanes and arylsulfonyl azides via Path b (Fig. 8 ) was not possible. Fig. 8: Proposed reaction mechanism. Cycloaromatization of vinylsilanes with arylsulfonylazides via Path a and Path b. Full size image In conclusion, we have reported a photoredox-catalyzed cycloaromatization of ortho -alkynylaryl vinylsilanes and arylsulfonyl azides, furnishing naphthyl-fused benzosilole skeletons with wide functional group tolerance. This protocol features a unique combination of cascade S-N/C-S bond cleavages and α-silyl radical Smiles rearrangement. 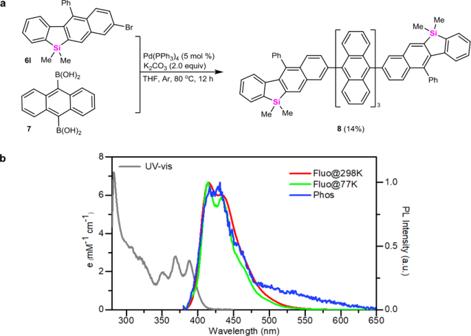Fig. 6: Synthetic applications of this method. aSynthesis of π-conjugated teranthracene-tethered 1-phenyl-2,3-benzosilafluorene8.bUV-vis absorption and PL spectra of benzosilafluorene8measured in diluted toluene solution (10−5M) (a.u. refers to the arbitrary unit. Fluo@298K refers to the fluorescence spectra measured at 298 K. Fluo@77K refers to the fluorescence spectra measured at 77 K. Phos refers to the phosphorescence spectra.). 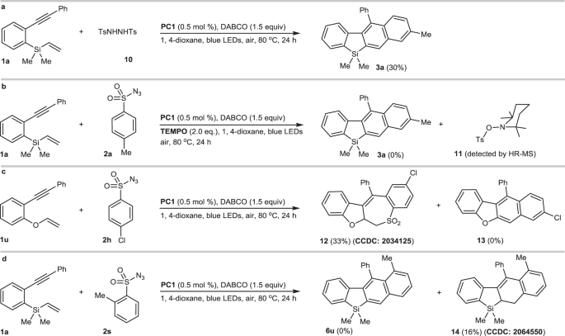Fig. 7: Preliminary mechanism studies. aPhotocatalyzed cycloaromatization of vinylsilane1awith sulfonylhydrazine10.bRadical intermediate trapping reaction by TEMPO.cPhotocatalyzed coupling-cyclization of vinylether1uwith arylsulfonylazide2h.dPhotocatalyzed coupling-cyclization of vinylsilane1awithortho-methylphenylsulfonyl azide2s. 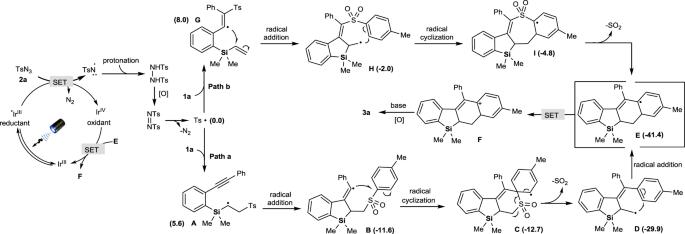Fig. 8: Proposed reaction mechanism. Cycloaromatization of vinylsilanes with arylsulfonylazides via Path a and Path b. These silaarenes show promising potential in luminescent materials, and further application studies of these highly π-conjugated siloles in luminescent materials are undergoing in our lab. Procedure for the photocatalyzed cycloaromatization of vinylsilanes with arylsulfonylazides To a 10 mL vial equipped with a magnetic stir bar, was added vinylsilanes 1 (0.2 mmol), arylsulfonylazides 2 (0.8 mmol), DABCO (33 mg, 0.3 mmol), [Ir{dt(tBu) 2 ppy} 2 (dtbbpy)][PF 6 ] PC1 (1.3 mg, 0.5 mol %) and 1,4-dioxane (2.0 mL) under air conditions. The vial was equipped with a Teflon septum and stirred at 80 °C under blue LED irradiation with two Kessil LEDs (30 W, 456 nm, ~3 cm away from the reaction mixture) for 24 h. The solvent was removed in vacuo and the residue was purified by flash column chromatography on silica gel to yield the desired products.